Multifunctional evolution of B andAGL6MADS box genes in orchids 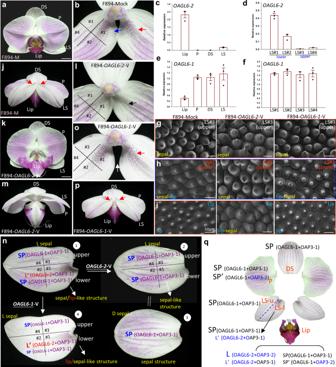Fig. 1: The emergence of L’ and SP’ complexes in orchid flowers revealed modified protein interactions in the P-code model. aA flower of wild-type control (mock)PhalaenopsisF894. LP lips, P petals, DS dorsal sepals, LS lateral sepals. Bars = 15 mm.bClose-up of the lateral sepals from (a), which are divided into a lower part (#1, 2) and an upper part (#3, 4). The red spots (red arrow) and curved edge (blue arrow) were observed in portion #1.c–fThe expression ofOAGL6-2(c) andOAGL6-1(e) in lips (Lip), petals (P), dorsal sepals (DS) and lateral sepals (LS). The expression ofOAGL6-2(d) andOAGL6-1(f) in four parts of lateral sepals. Error bars show ±SEM,n= 3 biologically independent samples.gThe epidermal cells of the #3 portion in the upper lateral sepals of wild-type control (mock) (left),OAGL6-2-VIGS (middle) andOAGL6-1-VIGS (right) F894 flowers showing conical cell morphology. Bar = 50 µm.hThe epidermal cells of the #1 portion in lower lateral sepals of wild-type control (left) andOAGL6-1-VIGS (right) flowers exhibit a flattened sepal/lip-like cell morphology, whereas those ofOAGL6-2-VIGS (middle) F894 exhibits conical cell morphology. Bar = 50 µm.iThe epidermal cells of the wild-type control (left) andOAGL6-1-VIGS (right) lips exhibit a flattened lip-like cell morphology, whereas those ofOAGL6-2-VIGS (middle) F894 exhibit conical cell morphology. Bar = 50 µm. In (g,h,i), each experiment was repeated twice independently with similar results.jBack view of the lateral sepals from (a), which show curved edges in the lower portion (red arrow).kA flower ofOAGL6-2-VIGSPhalaenopsisF894. Bars = 15 mm.lClose-up of the lateral sepals from (k), which show flattened edges without red spots (arrow) in portion #1.mBack view of the lateral sepals from (k), which show flattened edges in the lower portion (circle).nSummary of the protein interactions in four different parts of the lateral sepals of wild-type control (-1),OAGL6-2-VIGS (-2), andOAGL6-1-VIGS (-4) F894 as well as dorsal sepals of wild-type control (-3). In the wild-type control (-1), the upper lateral (L) sepals have only SP complex (OAGL6-1 + OAP3-1 + OPI) function, whereas the lower lateral sepals have both high SP (OAGL6-1 + OAP3-1 + OPI) and low L’ (OAGL6-2 + OAP3-1 + OPI) complex functions, and they are converted to a sepal/lip-like structure. InOAGL6-2-VIGS (-2), both the upper and lower lateral (L) sepals have only SP complex (OAGL6-1 + OAP3-1 + OPI) function, and the whole lateral sepals are converted into a dorsal sepal-like structure (-3), which has only SP complex (OAGL6-1 + OAP3-1 + OPI) activity. InOAGL6-1-VIGS (-4), the upper lateral (L) sepals have only SP complex (OAGL6-1 + OAP3-1 + OPI) function, whereas the lower lateral sepals have low SP (OAGL6-1 + OAP3-1 + OPI) and high L’ (OAGL6-2 + OAP3-1 + OPI) complex functions, and they are converted to a more lip/sepal-like structure.oClose-up of the lateral sepals of anOAGL6-1-VIGSPhalaenopsisF894 flower. The red spots (red arrow) and enhanced curved edge (white arrow) were observed in portion #1.pBack view of the lateral sepals from (o), which show curved edges in the lower portion (red arrow).qSummary of the modified P-code protein interactions in orchid flowers. The dorsal and upper parts of the lateral sepals (LS-u) are exclusively regulated by the SP complex (OAGL6-1 + OAP3-1). The lower part of the lateral sepal (LS-l) is regulated by a strong SP complex (OAGL6-1 + OAP3-1) and a weak L’ complex (OAGL6-2 + OAP3-1). The petals (P) are regulated by both SP (OAGL6-1 + OAP3-1) and SP’ (OAGL6-1 + OAP3-2) complexes. The lips (Lip) are primarily regulated by the L complex (OAGL6-2 + OAP3-2) and, to a small degree, by the L’/SP/SP’ complexes. Source data underlying Fig. 1c–f are provided as a Source Data file. We previously found that B and AGL6 proteins form L (OAP3-2/OAGL6-2/OPI) and SP (OAP3-1/OAGL6-1/OPI) complexes to determine lip/sepal/petal identities in orchids. Here, we show that the functional L’ (OAP3-1/OAGL6-2/OPI) and SP’ (OAP3-2/OAGL6-1/OPI) complexes likely exist and AP3 / PI/AGL6 genes have acquired additional functions during evolution. We demonstrate that the presumed L’ complex changes the structure of the lower lateral sepals and helps the lips fit properly in the center of the flower. In addition, we find that OAP3-1/OAGL6-1/OPI in SP along with presumed SP’ complexes regulate anthocyanin accumulation and pigmentation, whereas presumed L’ along with OAP3-2/OAGL6-2/OPI in L complexes promotes red spot formation in the perianth. Furthermore, the B functional proteins OAP3-1/OPI and OAGL6-1 in the SP complex could function separately to suppress sepal/petal senescence and promote pedicel abscission, respectively. These findings expand the current knowledge behind the multifunctional evolution of the B and AGL6 genes in plants. In flowering plants, the four whorls of flower organs are regulated by the interaction of four classes of homeotic genes based on the ABCE model [1] , [2] , [3] , [4] , [5] . In angiosperms, B class proteins consist of two clades, APETALA3 (AP3)- and PISTILLATA (PI)-like proteins, which have been mainly found to control petal and stamen identity [6] , [7] , [8] , [9] . AP3/PI heterodimers could further interact with A/E- and C/E-function proteins to form higher-order heterotetrameric complexes in regulating petal and stamen development [6] , [10] , [11] , [12] , [13] . In addition to regulate floral organ identity1 [6] , [14] , [15] , [16] , A/E-class AGL6 gene has been found to control meristem identity and ovule development [14] , [15] , [17] , [18] , [19] . However, whether AP3 / PI/AGL6 have evolved additional functions in different plant species during evolution remains unknown. Based on the conserved principle of the perianth (P) code in orchids, the higher-order SP complex (OAP3-1/OAGL6-1/OAGL6-1/OPI) specifies sepal/petal identity, whereas the L complex (OAP3-2/OAGL6-2/OAGL6-2/OPI) is exclusively required for lip formation [6] . Since the L complex gene OAGL6-2 is also expressed in lateral sepals whereas OAP3-2 is also expressed in petals [6] , these genes may have other, still unknown roles in determining the morphological identity of lateral sepals or petals beyond the P code. Furthermore, L and SP complex genes are continuously expressed throughout flower development [6] , suggesting that OAP3 , OPI and OAGL6 may have additional functions during organ morphogenesis. To uncover these questions, we used virus-induced gene silencing (VIGS)-based gene knockdown to comprehensively functionally characterize the genes from the L and SP complexes and their target networks in Phalaenopsis orchids. Here, we show the existence of L′ (OAP3-1/OAGL6-2/OPI) and SP’ (OAP3-2/OAGL6-1/OPI) complexes. The L′ complex has the function in regulating the structure of the lower part of the lateral sepals and helps the lips fit properly in the center of the flower. We also find that B and AGL6 proteins in P-code harbor additional function during orchid flower development. OAP3-1/OAGL6-1/OPI in SP complexes regulate anthocyanin accumulation and pigmentation whereas OAP3-2/OAGL6-2/OPI in L complexes promotes red spot formation in the perianth. Furthermore, SP complex proteins OAGL6-1 is found to be able to promote pedicel abscission whereas OAP3-1/OPI could function to suppress sepal/petal senescence. The finding of L′/SP′ complexes in the advanced P code OAGL6 -2 in the L complex is not only highly expressed in the lip but also expressed at a very low level in the lateral sepals of orchid flowers [6] (Fig. 1a–c ). OAGL6-2 is mainly expressed in the lower part of the lateral sepals in different Phalaenopsis varieties (Fig. 1d ) (Supplementary Fig. 1a–o ) and in various species of orchids (Supplementary Fig. 2a–r ), whereas the SP complex-associated gene OAGL6-1 is expressed evenly in all parts of the lateral sepals (Fig. 1e, f ) (Supplementary Fig. 1p–t ). Interestingly, OAGL6-2 -VIGS not only caused the conversion of the lip into a petal-like structure (Fig. 1k ) but also caused the loss of the distinct characteristics such as red spots or a greenish color (Fig. 1b ) (Supplementary Fig. 1b, e, h, k, n ) and the curved edge (Fig. 1b, j ) (Supplementary Fig. 1x ) on the lower part of the lateral sepals (Fig. 1l, m ) (Supplementary Fig. 1y ). In addition to converting lip cells into upper sepal epidermal cells (Fig. 1i , middle) (Supplementary Fig. 1w , middle), the epidermis in OAGL6-2 -VIGS lower lateral sepals (Fig. 1h , middle) (Supplementary Fig. 1v , middle) was clearly converted into upper sepal epidermis (Fig. 1g , left and middle) (Supplementary Fig. 1u , left and middle). This result indicated that OAGL6-2 must function in determining lower lateral sepal identity. Fig. 1: The emergence of L’ and SP’ complexes in orchid flowers revealed modified protein interactions in the P-code model. a A flower of wild-type control (mock) Phalaenopsis F894. LP lips, P petals, DS dorsal sepals, LS lateral sepals. Bars = 15 mm. b Close-up of the lateral sepals from ( a ), which are divided into a lower part (#1, 2) and an upper part (#3, 4). The red spots (red arrow) and curved edge (blue arrow) were observed in portion #1. c – f The expression of OAGL6-2 ( c ) and OAGL6-1 ( e ) in lips (Lip), petals (P), dorsal sepals (DS) and lateral sepals (LS). The expression of OAGL6-2 ( d ) and OAGL6-1 ( f ) in four parts of lateral sepals. Error bars show ±SEM, n = 3 biologically independent samples. g The epidermal cells of the #3 portion in the upper lateral sepals of wild-type control (mock) (left), OAGL6-2 -VIGS (middle) and OAGL6-1 -VIGS (right) F894 flowers showing conical cell morphology. Bar = 50 µm. h The epidermal cells of the #1 portion in lower lateral sepals of wild-type control (left) and OAGL6-1 -VIGS (right) flowers exhibit a flattened sepal/lip-like cell morphology, whereas those of OAGL6-2 -VIGS (middle) F894 exhibits conical cell morphology. Bar = 50 µm. i The epidermal cells of the wild-type control (left) and OAGL6-1 -VIGS (right) lips exhibit a flattened lip-like cell morphology, whereas those of OAGL6-2 -VIGS (middle) F894 exhibit conical cell morphology. Bar = 50 µm. In ( g , h , i ), each experiment was repeated twice independently with similar results. j Back view of the lateral sepals from ( a ), which show curved edges in the lower portion (red arrow). k A flower of OAGL6-2 -VIGS Phalaenopsis F894. Bars = 15 mm. l Close-up of the lateral sepals from ( k ), which show flattened edges without red spots (arrow) in portion #1. m Back view of the lateral sepals from ( k ), which show flattened edges in the lower portion (circle). n Summary of the protein interactions in four different parts of the lateral sepals of wild-type control (-1), OAGL6-2 -VIGS (-2), and OAGL6-1 -VIGS (-4) F894 as well as dorsal sepals of wild-type control (-3). In the wild-type control (-1), the upper lateral (L) sepals have only SP complex (OAGL6-1 + OAP3-1 + OPI) function, whereas the lower lateral sepals have both high SP (OAGL6-1 + OAP3-1 + OPI) and low L’ (OAGL6-2 + OAP3-1 + OPI) complex functions, and they are converted to a sepal/lip-like structure. In OAGL6-2 -VIGS (-2), both the upper and lower lateral (L) sepals have only SP complex (OAGL6-1 + OAP3-1 + OPI) function, and the whole lateral sepals are converted into a dorsal sepal-like structure (-3), which has only SP complex (OAGL6-1 + OAP3-1 + OPI) activity. In OAGL6-1 -VIGS (-4), the upper lateral (L) sepals have only SP complex (OAGL6-1 + OAP3-1 + OPI) function, whereas the lower lateral sepals have low SP (OAGL6-1 + OAP3-1 + OPI) and high L’ (OAGL6-2 + OAP3-1 + OPI) complex functions, and they are converted to a more lip/sepal-like structure. o Close-up of the lateral sepals of an OAGL6-1 -VIGS Phalaenopsis F894 flower. The red spots (red arrow) and enhanced curved edge (white arrow) were observed in portion #1. p Back view of the lateral sepals from ( o ), which show curved edges in the lower portion (red arrow). q Summary of the modified P-code protein interactions in orchid flowers. The dorsal and upper parts of the lateral sepals (LS-u) are exclusively regulated by the SP complex (OAGL6-1 + OAP3-1). The lower part of the lateral sepal (LS-l) is regulated by a strong SP complex (OAGL6-1 + OAP3-1) and a weak L’ complex (OAGL6-2 + OAP3-1). The petals (P) are regulated by both SP (OAGL6-1 + OAP3-1) and SP’ (OAGL6-1 + OAP3-2) complexes. The lips (Lip) are primarily regulated by the L complex (OAGL6-2 + OAP3-2) and, to a small degree, by the L’/SP/SP’ complexes. Source data underlying Fig. 1c–f are provided as a Source Data file. Full size image How can OAGL6-2 function in determining lower lateral sepal identity without the presence of its L complex partner OAP3-2? Is it possible that OAGL6-2 interacts with OAP3-1 in the SP complex to form a new L′ complex (OAGL6-2 + OAP3-1) that has a similar function as the L complex? To test this assumption, a FRET analysis for orchid proteins was performed in tobacco leaf cells [1] , [9] . The result indicated that the OAGL6-2 could not only form a L complex (OAGL6-2 + OAP3-2 + OPI) (Supplementary Fig. 3a ) but also likely interacts with OAP3-1 in the SP complex to form a new L′ complex (OAGL6-2 + OAP3-1) (Supplementary Fig. 3b ). Thus, the lower lateral sepals likely have both high SP (OAGL6-1 + OAP3-1+OPI) and low L′ (OAGL6-2 + OAP3-1 + OPI) complex functions (Fig. 1n-1 ). In OAGL6-2 -VIGS, the reduced OAGL6 -2 in the lower lateral sepals likely caused reduced L′ complex activity and proportionally increased SP complex activity, resulting in a more upper lateral sepal structure/morphology (Fig. 1n-2 ) and turning the whole lateral sepals to a nearly identical dorsal sepal structure (Fig. 1n-3 ). Fig. 2: The SP/SP’ complexes regulated pigmentation, and the L/L’ complexes regulated red spot formation in orchid flowers. a–e Flowers ( a ), dorsal sepals ( b ), lateral sepals ( c ), petals ( d ) and lips ( e ) of wild-type control (Mock), PeMYB12 -VIGS, OAGL6-1 -VIGS, OAP3-1 -VIGS, OPI -VIGS, PeMYB11 -VIGS, OAGL6-2 -VIGS and OAP3-2 -VIGS Phalaenopsis F894 flowers. f – h The expression of PeMYB12 in the lips (Lip), petals (P), dorsal sepals (DS) and lateral sepals (LS) of OAGL6-1 -VIGS ( f ), OAP3 -1 -VIGS ( g ) and OPI -VIGS ( h ) F894. Error bars show ± SEM. n = 3 biologically independent samples. i The detection of anthocyanin content in the lips (Lip), petals (P), dorsal sepals (DS) and lateral sepals (LS) of wild-type control (Mock), PeMYB12 -VIGS, OAP3-1 -VIGS, OAGL6-1 -VIGS and OPI -VIGS F894. Error bars show ±SEM. n = 3 biologically independent samples. The p value indicates significant differences from the control (Mock) value. The statistical test used was two-sided according to Student’s t -test. j Summary of the protein complexes regulating pigmentation and red spot formation in orchid flowers. The SP complex is exclusively required for the activation of PeMYB12 expression and anthocyanin accumulation in dorsal (DS) and lateral (LS) sepals. The SP and SP’ complexes have complementary functions in regulating anthocyanin accumulation in the petals (P) and lips (Lip). The L/L’ complexes control PeMYB11 expression and spot formation in the lower part of the lateral sepals and lips. k Close-up of the lower part of the lateral sepals from ( c ). The wild-type control (Mock) contained red spots (circle and red arrow) that were absent in PeMYB11 -VIGS and OAGL6-2 -VIGS (blue arrows). l The expression of PeMYB11 in the lips (Lip), petals (P), dorsal sepals (DS) and lateral sepals (LS) of OAGL6-2 -VIGS F894. The expression of PeMYB11 in lateral sepals (LS) is enlarged in the box. Error bars show ±SEM. n = 3 biologically independent samples. Source data underlying Figs. 2f–i and 2l are provided as a Source Data file. Full size image Fig. 3: The OAP3-1 and OPI B functional proteins regulated sepal/petal senescence. a – c The inflorescence ( a ), front view ( b ) and back view ( c ) of flowers of the control (Mock) Phalaenopsis F894. d – f The inflorescence ( d ), front view ( e ) and back view ( f ) of flowers of OAP3-1 -VIGS F894, which showed early senescence of the sepals (red arrows). g The senescence of the OAP3-1 -VIGS petal (white arrow) occurred later than did that of the dorsal/lateral sepals (red arrow). h – i The inflorescence ( h ) and front view ( i ) of flowers of OPI -VIGS F894, which showed early senescence of the sepals (red arrow) and petals (white arrow). j The dorsal (DS) and lateral (LS) sepals of control (Mock), OAGL6-1 -VIGS, OAP3-1 -VIGS, and OPI -VIGS F894 (from left to right) at the same stage. k Summary of the protein complexes that regulate sepal/petal senescence in orchid flowers. The OAP3-1/OPI B functional proteins may form a senescence complex (S), which is exclusively required for the suppression of PeSAG39/PeEDF1/2 expression and senescence in dorsal (DS) and lateral (LS) sepals. S and minor S’ (OAP3-2/OPI) complexes have complementary functions in regulating petal (P) senescence. l – n At the same stage, all the flowers were senescent and abscised from the OAP3-1 -VIGS-late ( l , middle) ( m ) and OPI -VIGS-late ( l , right) ( n ) inflorescences, whereas the flowers of the control (Mock) inflorescences showed no sign of senescence or abscission ( l , left). o – p Analysis of the expression profile for OAP3-1/OPI/OAGL6-1 ( o ) and PeSAG39/PeEDF1/2 ( p ) throughout flower development. The dashed lines indicate that the senescence of the F894 flowers starts at 80–90 days after flower opening. Error bars show ±SD. n = 3 biologically independent samples. q , r Analysis of the expression of OAP3-1/OPI/OAGL6-1 ( q ) and PeSAG39/PeEDF1/2 ( r ) in the petals (P), dorsal sepals (DS) and lateral sepals (LS) of control (Mock), OAP3-1 -VIGS-late and OPI -VIGS-late F894 flowers. Error bars show ±SEM. n = 3 biologically independent samples. Source data underlying Fig. 3o–r are provided as a Source Data file. Full size image In the OAGL6-1 -VIGS flowers, only the structure/morphology of the lower lateral sepals was affected (Fig. 1o ), in which SP complex activity was reduced and in which the proportion of the L′ complex increased (Fig. 1n-4 ), resulting in a flatter lip-like epidermis in the lower lateral sepals (Fig. 1h-3 ) (Supplementary Fig. 1v - 3 ) with an enhanced curvature of the edge (Fig. 1o, p ) (Supplementary Fig. 1z ). FRET analysis showed that OAGL6-1 could not only form an SP complex with OAP3-1 (Supplementary Fig. 3c ) but also interacts with OAP3-2 (an L complex component) to form the SP’ complex (OAGL6-1 + OAP3-2 + OPI) (Supplementary Fig. 3d ). Fig. 4: The OAGL6-1 protein regulated pedicel abscission in orchids. a , b The flowers were senescent and abscised completely from the control (Mock) inflorescence ( a ), whereas senescent flowers were not abscised from the OAGL6-1 -VIGS inflorescence ( b ) of Phalaenopsis V3. c The senescent flowers were still not abscised three months after the plant ( b ) had completely dried. d – f The back views of flowers of the control (Mock) ( d ) and OAGL6-1 -VIGS ( e ) Phalaenopsis V3. A dark brown color was observed in the pedicel of OAGL6-1 -VIGS (red arrow in ( e , f )) but was absent in the control (Mock) pedicel (blue arrow in ( d )) ( f ). g – h The longitudinal views for pedicels (ped) and the connected stems of the control (Mock) ( g) and OAGL6-1 -VIGS V3 ( h ) after staining by phloroglucinol. The arrows indicate the AZ in the junction of the pedicel and stem. The dashed lines indicate the place used for the cross view in ( i , j ). Bars = 1 mm. i Cross view of the pedicels of the control (Mock), OAP3-1 -VIGS and OAGL6-1 -VIGS V3 (from left to right) after staining by phloroglucinol. Bars = 1 mm. j Close-up image of the phloroglucinol-stained pedicels from ( i ). Bars = 100 µm. k , n Analysis of the expression levels of PeVND1 , PeMYB85 , PeMYB46 , and PeMYB63 ( k ) as well as PeBOP1 and PeBOP2 ( n ) in the pedicels of control (Mock) and OAGL6-1 -VIGS V3 flowers. Error bars show ±SEM. n = 3 biologically independent samples. The p value indicates significant differences from the control (Mock) value. The statistical test used was two-sided according to Student’s t -test. l , m SEM image of pedicel AZs in control (Mock) ( l ) and OAGL6-1 -VIGS ( m ) V3 flowers. Bars = 50 µm. o , p Close-up of the phloroglucinol-stained junctions for the pedicel (ped) and the stem of the control (Mock) ( o ) and OAGL6-1 -VIGS V3 ( p ) from ( g , h ). The arrows indicate the AZ region with the small differentiated cells formed. The cells in the AZ region in ( p ) were altered by the penetration of lignin from the pedicel to the stem. Bars = 300 µm. In ( j , l , m , o , p ), each experiment was repeated twice independently with similar results. q Analysis of the expression levels of OAP3-1 , OAP3-2 , OAGL6-1 , OAGL6-2 , and OPI in 15 mm and mature flower pedicels of control (Mock) and OAGL6-1 -VIGS V3 flowers. The data were derived from one NGS data. r In wild-type orchid flowers, OAGL6-1 proteins may form an abscission complex (A) to promote the abscission of pedicels by suppressing the expression of VND1/MYB46/63/85 and lignin formation and to ensure the normal BOP1/2 expression and subsequent AZ formation. Source data underlying Figs. 4k, 4n, and 4q are provided as a Source Data file. Full size image Our results revealed that OAGL6 proteins are the determining factors that form either the L or SP complex in controlling orchid perianth identity. OAGL6-1 determines SP (with OAP3-1) or SP′ (with OAP3-2) complexes, and OAGL6-2 determines L (with OAP3-2) or L′ (with OAP3-1) complexes. In orchid flowers (Fig. 1q ), the dorsal and upper parts of lateral sepals are exclusively regulated by the SP complex. The lower part of the lateral sepals showed a sepal/lip-like morphology since it was regulated by a strong SP complex and a weak L′ complex. Petals are regulated by both SP and SP’ complexes. The lips were regulated mainly by the L complex and weakly by L′/SP/SP′ complexes. One interesting question is why the L′ complex coexists with the SP complex in the lower lateral sepals of orchid flowers. We found that the flat lip-like epidermis (Fig. 1h-1 ) altered the structure/morphology and caused a curved edge in both lower lateral sepals (Fig. 1b, j, n-1 ) (Supplementary Fig. 1n, x ), which created space to fit the lip more properly in the center, without being too prominent (Fig. 1b, j ). Thus, the production of the lips should have coevolved with the emergence of the L′ complex in the lower lateral sepals during orchid flower evolution. This structural change does not occur in the dorsal sepals since their position in the flower does not affect the development of the lips. The SP/SP’ complexes regulate pigmentation in the perianth A complete reduction of full-red pigmentation in the dorsal/lateral sepals was observed in OAGL6-1 -VIGS (Fig. 2a, b, c , left 3), OAP3-1 -VIGS (Fig. 2a, b, c , left 4) and OPI -VIGS (Fig. 2a, b, c , left 5) F894 flowers compared with the Phalaenopsis F894 control flowers (Fig. 2a, b, c , left 1), and this pigmentation was similar to that observed in PeMYB12 -VIGS F894 plants (Fig. 2a, b, c , left 2). A significant downregulation of PeMYB12 , which has been reported to regulate flower pigmentation and anthocyanin accumulation [20] , [21] , [22] , [23] , [24] , [25] , [26] , was observed in the dorsal/lateral sepals of OAGL6-1 -VIGS (Fig. 2f ), OAP3-1 -VIGS (Fig. 2g ) and OPI -VIGS (Fig. 2h ) F894 flowers. The level of anthocyanins was clearly reduced in the OAGL6-1 -VIGS, OAP3-1 -VIGS F894 and OPI -VIGS dorsal/lateral sepals, similar to that in the PeMYB12 -VIGS F894 flowers (Fig. 2i ). Since only OAGL6-1 , OAP3-1 and OPI in SP complex expressed in the dorsal/lateral sepals, indicating that the SP complex (OAGL6-1 + OAP3-1 + OPI) is exclusively required for anthocyanin accumulation in dorsal/lateral sepals by activating the PeMYB12 expression (Fig. 2j ). Silencing of either OAGL6-1 , OAP3-1 or OPI expression caused the same disruption of the SP complex and the reduction in pigmentation in dorsal/lateral sepals (Fig. 2b, c , left 3 to 5). In contrast, silencing of OAGL6-2 or OAP3-2 expression in the L complex did not affect the pigmentation (Fig. 2a, b, c , left 7 and 8) in the dorsal/lateral sepals. Different from that observed in dorsal/lateral sepals, a significant and relative weak reduction in full-red pigmentation, downregulation of PeMYB12 expression and accumulation of anthocyanins in petals was observed in OAGL6-1 -VIGS (Fig. 2d , left 3, f, i) and OPI -VIGS F894 flowers (Fig. 2d , left 5, h, i) and not in OAP3-1 -VIGS (Fig. 2d , left 4, g, i) or OAP3-2 -VIGS (Fig. 2d , left 8) F894 flowers. This result indicated that silencing of OAP3-1 or OAP3-2 expression caused the disruption of only the function of either the SP or SP’ complex and had no or very weak effect on the reduction in pigmentation in the petals (Fig. 2d , left 4 and 8). This result actually supported the coexistence of SP and SP’ complexes in petals, which have complementary functions in regulating both petal identity and pigmentation (Figs. 1 q, 2j ). Silencing of OAGL6-1 (Fig. 2e , left 3), OAP3-1 (Fig. 2e , left 4), OPI (Fig. 2e , left 5) and OAP3-2 (Fig. 2e , left 8) caused a similar weaker reduction in full-red pigmentation, PeMYB12 expression (Fig. 2f, g, h ) and anthocyanin accumulation (Fig. 2i ) in the lips than did the silencing of PeMYB12-VIGS (Fig. 2e , left 2, 2i). This result revealed that SP and SP’ complexes are involved in the regulation of anthocyanin accumulation in the lips, although to different degrees (Fig. 2j ). We also examined the VIGS of Phalaenopsis KA38501, which has yellow/red-orange perianth pigmentation (Supplementary Fig. 4a , top/left). Similar to PeMYB12 -VIGS KA38501 flowers (Supplementary Fig. 4a , top/middle and top/right), a reduction in red-orange pigmentation and anthocyanin content in the dorsal/lateral sepals of OAGL6-1/OAP3-1/OPI -VIGS KA38501 (Supplementary Fig. 4a , bottom, b, c, e) and in the flower petals of OAGL6-1/OPI -VIGS KA38501 (Supplementary Fig. 4a , bottom/left, bottom/right, d, e), as well as a relatively weak effect on lips of OAGL6-1/OAP3-1/OPI -VIGS KA38501 (Supplementary Fig. 4a, e ) flowers, were observed. These results strongly support that SP and SP’ complexes are involved in the regulation of anthocyanin accumulation and pigmentation in the orchid perianth. The L′ complex regulates red spot formation In addition to causing the conversion of lips to sepal/petal-like structures (Fig. 2a, e , left 7), OAGL6-2 -VIGS also resulted in a significant reduction in red spots (Fig. 2k , left) in the lateral sepals (Figs. 1 l, 2c , left 7, k, right), similar to that observed in PeMYB11 -VIGS (Fig. 2c , left 6, k, middle) Phalaenopsis F894 flowers. Interestingly, similar to that which occurred in OAGL6-2 (Fig. 1c ), PeMYB11 was also exclusively expressed in the lips (high) and lateral sepals (low) (Fig. 2l ), and its expression was significantly downregulated in the OAGL6-2 -VIGS flowers (Fig. 2l ). This result revealed that OAGL6-2 formed an L′ complex with OAP3-1 in the lateral sepals; in turn, this complex controls the activation of PeMYB11 (Fig. 2j ), which has been thought to be associated with red spot formation [22] , [27] . Silencing OAGL6-2 caused a severe reduction in L′ complex function, subsequently downregulating PeMYB11 expression (Fig. 2l ) and reducing red spot formation (Fig. 2c , left 7, k, right). Since OAP3-1 was expressed at a much higher level than OAGL6-2 was in the lateral sepals, the reduced amount of OAP3-1 in the OAP3-1 -VIGS lateral sepals is still able to form enough numbers of L′ complexes with a low amount of OAGL6-2 , with no effect on the red spot formation (Fig. 2c , left 4). This result supported that OAGL6-2 is the major component in the formation of L/L′ complexes in the control of PeMYB11 expression in lateral sepal and lips (Fig. 2j ). Red spot formation was not affected in the OAGL6-1 -VIGS lateral sepals (Fig. 2c , left 3, 1o), indicating the SP complex is not involved in regulating this process (Fig. 2j ). OAP3-1 and OPI suppress senescence of sepals/petals In addition to see the alteration in pigmentation, significantly earlier senescence for the dorsal/lateral sepals compared with that of the control (Fig. 3a–c ) was observed for the OAP3-1 -VIGS (Fig. 3d–f ) F894 flowers. In the controls, the senescence of the sepals and petals occurred simultaneously. The senescence of the OAP3-1 -VIGS petals occurred later than that of the dorsal/lateral sepals (Fig. 3d–f ), although it occurred earlier than that of the control F894 petals (Fig. 3g ). Similar early senescence for both dorsal/lateral sepals and petals was observed in OPI -VIGS flowers (Fig. 3h–j ). This early senescence phenotype was not observed in OAGL6-1 -VIGS (Fig. 3j ), OAP3-2 -VIGS or OAGL6-2 -VIGS flowers. These results indicated that only the B class proteins (OAP3-1 + OPI) from the SP complex may form an independent senescence-associated complex (S complex) in suppressing sepal/petal senescence in orchids (Fig. 3k ). Since the senescence of the petals occurred later than that of the sepals in OAP3-1 -VIGS flowers (Fig. 3d–f ), OAP3-2+OPI from the SP′ complex might form an S’ complex in petals with a complementary function in suppressing petal senescence with the SP complex, albeit in a weaker manner (Fig. 3k ). To avoid any influence on flower senescence due to the alteration of flower organ identity in VIGS of OAP3-1/OPI , a VIGS experiment was performed by late infection after flower organs were evaluated during the later stage (VIGS-late). When all the flowers were senescent and had abscised from the OAP3-1 -VIGS-late (Fig. 3l, m ) or OPI -VIGS-late (Fig. 3l, n ) F894 inflorescences, the flowers of the control inflorescences did not yet show senescence (Fig. 3l ). A similar early senescence phenotype was also observed in the OAP3-1 -VIGS-late and OPI -VIGS-late V3 (Supplementary Fig. 5 ) and KA38501 (Supplementary Fig. 6 ) Phalaenopsis flowers. This result supports that orchid B class proteins (OAP3-1 + OPI) suppress the senescence of sepals/petals (Fig. 3k ). In wild-type F894, flower senescence starts at 80–90 days after flower opening (AFO). Interestingly, OAP3-1/OPI expression starts to decrease at 80 days AFO and is continuously downregulated afterward to a basal level until flower senescence is complete at 110 days AFO (Fig. 3o ). In contrast, an opposite expression pattern, starting to increase at 80 days AFO until reaching the highest level at 110 days AFO, was observed for the senescence-associated gene PeSAG39 [28] and for downstream genes involved in ethylene signaling ( PeEDF1/ 2) [29] , [30] , [31] (Fig. 3p ). A similar downregulation of OAP3-1/OPI (Fig. 3q ) and upregulation of PeSAG39/PeEDF1/2 (Fig. 3r ) was observed in the sepals/petals of both OAP3-1 -VIGS-late and OPI -VIGS-late flowers. A similar gene expression profiles were also observed in the OAP3-1 -VIGS-late and OPI -VIGS-late V3 (Supplementary Fig. 5 ) and KA38501 (Supplementary Fig. 6 ) Phalaenopsis flowers. These results support that OAP3-1 and OPI function in suppressing orchid flower senescence by negatively regulating PeSAG39/PeEDF1/2 . The expression of OAGL6-1 continuously increased 90 days AFO (Fig. 3o ) during flower development, which is opposite that of OAP3-1/OPI , and OAGL6-1 expression only slightly decreased or even increased in OAP3-1/OPI -VIGS-late senescent flowers (Fig. 3q ), respectively, further supporting that OAGL6 -1 in the SP complex is not involved in the regulation of orchid flower senescence. OAGL6-1 regulates the abscission of pedicels A significant defect in abscission of the pedicel was observed in OAGL6-1 -VIGS Phalaenopsis V3 (Fig. 4b, c ) and F894 (Supplementary Fig. 7a ) flowers. In contrast to the flowers of the control plants (Fig. 4a ) (Supplementary Fig. 7b ), all the senescent OAGL6-1 -VIGS flowers remained attached to the inflorescence (Fig. 4b ) (Supplementary Fig. 7a ), even after the plants were completely dry and had died (Fig. 4c ). A darker brown color in the pedicel of OAGL6-1 -VIGS Phalaenopsis V3 (Fig. 4e, f ) and F894 (Supplementary Fig. 7a, c, d, f ) flowers than in the control flowers (Fig. 4d, f ) (Supplementary Fig. 7e, f ) was observed. When the pedicel was treated with phloroglucinol staining, which turns lignin a dark red color [32] , a significantly darker red color was observed in the pedicels of OAGL6-1 -VIGS Phalaenopsis V3 (Fig. 4h, i, j , right) and F894 (Supplementary Fig. 7g ) flowers than in the control flowers (Fig. 4g, i, j , left) (Supplementary Fig. 7g ) and the OAP3-1 -VIGS (Fig. 4i, j , middle) (Supplementary Fig. 7g ) pedicel. The strong lignin formation in the OAGL6-1 -VIGS Phalaenopsis V3 pedicel was further confirmed by the strong yellow color staining by Auramine O (Supplementary Fig. 8a, b ). This dark red or yellow color for lignin staining clearly extended throughout the pedicel and ran through into the stem of the OAGL6-1 -VIGS Phalaenopsis V3 (Fig. 4h , Supplementary Fig. 8b ). In contrast, no dark red or yellow color for lignin staining was observed throughout the pedicel until the junction of the stem in the control flower (Fig. 4g , Supplementary Fig. 8a ). Furthermore, the expression levels of the secondary wall NAC master switch PeVND1 , the secondary wall MYB master switch PeMYB46 and the lignin-specific activator PeMYB63/85 (involved in the lignin biosynthetic pathway) [33] , [34] , [35] , [36] , [37] , [38] , [39] were significantly upregulated in the pedicel of OAGL6-1 -VIGS flowers (Fig. 4k ) (Supplementary Fig. 7h ). In the control abscised pedicel, a fully developed abscission zone (AZ) with cells displaying a fully rounded, intact appearance was observed (Fig. 4l ) (Supplementary Fig. 7i ). In contrast, upon manual pedicel removal from the senescent flower, broken cells at the fracture plane and a flattened cavity were observed in the OAGL6-1 -VIGS pedicel AZs (Fig. 4m ). The expression levels of PeBOP1 / 2 , which are necessary for the formation of the floral AZ [40] , [41] , were significantly downregulated in the OAGL6-1 -VIGS pedicel (Fig. 4n ) (Supplementary Fig. 7j ). Further analysis indicated that small differentiated cells that formed in the AZ of the control flower pedicel (Fig. 4o , Supplementary Fig. 8c, e ) were also observed in the junction of the pedicel and stem in the OAGL6-1 -VIGS pedicel (Fig. 4p , Supplementary Fig. 8d ); however, their formation was clearly altered by the penetration of lignin throughout the pedicel to the stem (Fig. 4p , Supplementary Fig. 8d, f ). These results revealed that the defect in abscission of the OAGL6-1 -VIGS pedicel was likely due to the strong increase in lignin formation in the pedicel, which tightly connected the pedicel to the stem and subsequently prevented the abscission of the pedicel from the stem. During this process, AZ was likely formed, although its further development and function were altered. When the expression levels of all the P-code genes in the pedicels were analyzed, the expression levels were OAGL6-1 (SP) = OPI (SP, L) > OAP3-1 (SP) > OAGL6-2 (L), and expression was not detected for OAP3-2 (L) (Fig. 4q ). Similar expression patterns for OAGL6-1 / OAP3-1/OAP3-2 were also observed in the pedicels of various species of orchids (Supplementary Fig. 9 ). Since defects in pedicel abscission were not observed in VIGS Phalaenopsis flowers with the silencing of the other P-code genes ( OAP3-1/OPI/OAGL6-2 / OAP3-2 ), OAGL6-1 is likely exclusively required for the regulation of pedicel abscission. Our results revealed that the OAGL6-1 protein has an additional function to ensure the final abscission of the pedicel through the downregulation of lignin formation and subsequent normal AZ development (Fig. 4r ). In the OAGL6-1 -VIGS pedicel, OAGL6-1 knockdown caused the upregulation of lignin biosynthetic genes and a high level of lignin in the pedicel, which altered AZ development and resulted in the strong blocking of pedicel abscission. B and AGL6 proteins form L (OAP3-2/OAGL6-2/OPI) and SP (OAP3-1/OAGL6-1/OPI) complexes to determine lip and sepal/petal identities in orchids [6] (Fig. 5 ). This study further showed the involvement of the proposed L′ complex (OAP3-1/OAGL6-2/OPI) in regulating the lower part of the lateral sepals and lip identity/morphology during orchid flower evolution to help the evolved lips fit properly in the center of the flowers (Fig. 5 ). In addition, the SP complex (OAP3-1/OAGL6-1/OPI) was found to regulate anthocyanin accumulation and pigmentation in sepals/petals, whereas an SP’ complex (OAP3-2/OAGL6-1/OPI) with the complementary function was identified in the petals (Fig. 5 ). L′/L complexes regulate the formation of red spots in the sepals/lips (Fig. 5 ). The roles of B and AGL6 genes in the regulation of flower color have never been experimentally verified in plants. We found that anthocyanin accumulation is correlated with LMYB12 but not LAGL6/LAP3/LPI expression in lily tepals (Supplementary Fig. 10 ), suggesting a possibly unique role for orchid OAGL6-1/OAP3-1/OPI in regulating flower pigmentation during evolution. Fig. 5: The multifunctional evolution of P-code genes in orchids. In orchids, two AGL6 ( OAGL6-1 , -2 ), two AP3 ( OAP3-1 , -2 ) and one PI ( OPI ) gene play key roles (blue dashed circle) in regulating perianth identity and other developmental processes in flowers. During early flower initiation, the L (OAP3-2/OAGL6-2/OPI) complex determines the lips, whereas the SP (OAP3-1/OAGL6-1/OPI) complex determines sepal/petal identity. In addition, an L’ complex (OAP3-1/OAGL6-2/OPI) is also likely involved in regulating the lips and lower parts of the lateral sepal identity/morphology, whereas an SP’ complex (OAP3-2/OAGL6-1/OPI) is likely involved in regulating the petal and lip identity/morphology. After flower organ identity has been determined, SP/SP’ complexes have an additional function in positively regulating (black arrow→) anthocyanin accumulation and pigmentation in sepals/petals, whereas L’/L complexes can regulate (red arrow→) red spot formation in lateral sepals and lips. During flower development, the OAP3-1/OPI B class proteins from the SP complex could form a separate senescence complex (S) to suppress ( ⊣ ) the senescence of the sepal/petal in orchids. An S’ complex (OAP3-2/OPI/X) with minor complementary function for the S complex could suppress ( ⊣ ) petal senescence. The orchid OAGL6-1 from the SP complex may form an abscission complex (A) to ensure (→) the abscission of the pedicel from senescent flowers during the late stage of flower development. AGL6-1: OAGL6-1, AGL6-2: OAGL6-2, AP3-1: OAP3-1, AP3-2: OAP3-2, PI: OPI. Full size image Unexpectedly, B functional OAP3-1 and OPI could function separately from SP complex in suppressing the senescence of the sepals/petals of orchids, whereas OAP3-2/OPI with complementary function to that of the OAP3-1/OPI is present in the petals (Fig. 5 ). The ability of AP3/PI orthologs to regulate flower organ senescence is surprising. A similar downregulation of AP3/PI expression during petal/tepal development/senescence was also observed in other various species of orchids (Supplementary Fig. 11 ), the dicot Arabidopsis and the monocot lily (Supplementary Fig. 12 ), revealing the possibly conserved role of AP3/PI orthologs in regulating flower senescence in flowering plants throughout evolution. The finding of the functions for B genes outside of floral organ identity specification is interesting. In addition to the orchid OAP3-1/OPI in this study, it has been reported that mutation in the apple B-function PI ortholog MdPI resulted in the production of parthenocarpic fruit [42] . Thus, evolutionary modification of the functions for the B class genes should occur and remains to be explored in more plant species. We found that OAGL6-1 in the SP complex also has additional features. The orchid OAGL6-1 could function to promote the abscission of the pedicel (Fig. 5 ). This function is clearly independent from that of the B proteins OAP3-1/OPI in the SP complex (Fig. 5 ). Since orchid flowers abscised from the pedicel, which is different from the process in plant species such as Arabidopsis and lily (in which abscission occurs from the base of the flower organs), OAGL6-1 orthologs may have evolved an additional expression pattern in the pedicel to control lignin levels during the evolution of this type of flower and to further develop this additional function to control pedicel abscission. Interestingly, it has been reported that two E-function SEP proteins (SLMBP21 and SEP4/J2) were involved in the regulation of pedicel abscission zone development in tomato [43] , [44] . Mutations in SLMBP21 or SEP4/J2 caused the lack of the abscission zone on the pedicels (jointless pedicels) of flowers [43] , [44] . However, the mechanism regulated by OAGL6-1 in orchids is clearly different from that for tomato SLMBP21 , since OAGL6-1 suppressed lignin levels in pedicels whereas SLMBP21 affected common meristem activity genes such as LeWUS and LATERAL SUPPRESSOR in the AZ [43] . In conclusion, a scenario was proposed to elucidate the evolutionary modification of the functions of the B class AP3 / PI and AGL6 genes. In the eudicot Arabidopsis , AP3/PI proteins form an SP-like complex with A/E proteins in regulating petal formation. In the monocots lily (Liliales) and orchid (Orchidaceae), the AP3/PI proteins specifically interact with the AGL6-like protein to form SP-like complexes in lily or SP/SP′L/L′ complexes in orchid to further regulate tepal (lily) or sepal/petal/lip (orchids) identity. AP3/PI proteins also likely evolved to have a conserved function in Arabidopsis , lily and orchid in regulating petal ( Arabidopsis ), tepal (lily) and sepal/petal (orchid) senescence. During orchid flower evolution, AP3/PI/AGL6 in SP/SP′/L/L′ complexes further developed a function involved in the specific regulation of pigmentation in the perianth, and AGL6-1 in the SP complex acquired an additional function in controlling pedicel abscission, which is absent in Arabidopsis and lily. Plant materials Species and cultivars of orchids used in this study, including the moth orchids ( Phalaenopsis Sogo Yukidian ‘V3’, P . F894, P . A09705, P . A09617, P . A07068, P . KA38501), Oncidium spp., Cymbidium spp., Dendrobium spp., Cattleya spp ., Brassocattleya spp., Neofinetia spp., Epidendrum spp., Paphiopedilum spp . (lady slipper orchids), were maintained in the greenhouse of National Chung-Hsing University, Taichung, Taiwan. Plants of Asiatic hybrid lilies ( Lilium spp .) used in this study were grown in the field in Houli, Taiwan. The Arabidopsis etr1-1 (CS237) Arabidopsis seeds were obtained from Dr. Long-Chi Wang, Department of Life Science, National Chung Hsing University, Taiwan. Real-time PCR analysis Quantitative real-time PCR was conducted using a Mini OpticonReal-Time PCR Detection System and Optical System Software version 3.0a (Bio-Rad Laboratories). For transcript measurements, the KAPA SYBR® FAST qPCRMaster Mix Universal (KAPA BIOSYSTEMS) was used. The amplification condition was one cycle at 95 °C for 1 min, followed by 40 cycles of 95 °C (for 15 s), 58 °C (for 15 s), and 72 °C (for 30 s), and plate reading after each cycle. The name and the sequence of the gene-specific primers for MADS box genes ( OAP3-1, OAP3-2, OAGL6-1, OAGL6-2, OPI ) of different orchids, PeMYB12, PeMYB11, PeSAG39, PeEDF1, PeEDF2, PeVND1, PeMYB85, PeMYB46, PeMYB63, PeBOP1 and PeBOP2 of orchids, LMYB12, LAGL6, LMADS1/LAP3, LMADS8/LPI, LMADS9/LPI of lily, AtAP3 and AtPI of Arabidopsis were listed in Supplementary Tables 1 to 2. The data were analyzed using CFX Manager TM Software (Version 3.0; Bio-Rad Laboratories, Inc.). 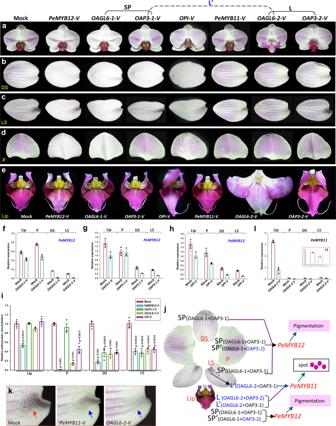Fig. 2: The SP/SP’ complexes regulated pigmentation, and the L/L’ complexes regulated red spot formation in orchid flowers. a–eFlowers (a), dorsal sepals (b), lateral sepals (c), petals (d) and lips (e) of wild-type control (Mock),PeMYB12-VIGS,OAGL6-1-VIGS,OAP3-1-VIGS,OPI-VIGS,PeMYB11-VIGS,OAGL6-2-VIGS andOAP3-2-VIGSPhalaenopsisF894 flowers.f–hThe expression ofPeMYB12in the lips (Lip), petals (P), dorsal sepals (DS) and lateral sepals (LS) ofOAGL6-1-VIGS (f), OAP3-1-VIGS (g) andOPI-VIGS (h) F894. Error bars show ± SEM.n= 3 biologically independent samples.iThe detection of anthocyanin content in the lips (Lip), petals (P), dorsal sepals (DS) and lateral sepals (LS) of wild-type control (Mock),PeMYB12-VIGS,OAP3-1-VIGS,OAGL6-1-VIGS andOPI-VIGS F894. Error bars show ±SEM.n= 3 biologically independent samples. Thepvalue indicates significant differences from the control (Mock) value. The statistical test used was two-sided according to Student’st-test.jSummary of the protein complexes regulating pigmentation and red spot formation in orchid flowers. The SP complex is exclusively required for the activation ofPeMYB12expression and anthocyanin accumulation in dorsal (DS) and lateral (LS) sepals. The SP and SP’ complexes have complementary functions in regulating anthocyanin accumulation in the petals (P) and lips (Lip). The L/L’ complexes controlPeMYB11expression and spot formation in the lower part of the lateral sepals and lips.kClose-up of the lower part of the lateral sepals from (c). The wild-type control (Mock) contained red spots (circle and red arrow) that were absent inPeMYB11-VIGS andOAGL6-2-VIGS (blue arrows).lThe expression ofPeMYB11in the lips (Lip), petals (P), dorsal sepals (DS) and lateral sepals (LS) ofOAGL6-2-VIGS F894. The expression ofPeMYB11in lateral sepals (LS) is enlarged in the box. Error bars show ±SEM.n= 3 biologically independent samples. Source data underlying Figs. 2f–i and 2l are provided as a Source Data file. The transcript levels for genes were determined using three replicates and were normalized using reference genes ACTIN for Phalaenopsis ( PACT4 ) [6] , [45] , [46] , α-tubulin for other orchids ( OnAT ) [6] , [47] , ACTIN for lily ( LilyACTIN ) [48] and UBQ10 for Arabidopsis ( At UBQ10 ) [49] (Supplementary Table 2 ). Anthocyanin content analysis Total anthocyanin content in the flower samples was determined according to the spectrophotometric method described previously [50] with slight modifications. Briefly, 100 mg of fresh flower tissues were homogenized in liquid nitrogen and added to 1 ml of 3 M HCl:H 2 O:MeOH (1:3:16, by volume). The crude extracts were agitated gently in the dark for 24 h at 4 °C and then centrifuged at 21,000 × g for 15 min. Anthocyanin levels in the supernatant were measured as A 530 – 0.24 A 653 by the spectrophotometer TECAN Infinite M200PRO with The i-control microplate reader software (Mannedorf, Switzerland) [51] . Phloroglucinol-HCl staining The junctions for the Phalaenopsis flower pedicel and stem were longitudinally cut, whereas 2-mm-thick Phalaenopsis pedicle slices were crossly cut from the base of the pedicel using a blade and put into 24-well plates. The staining solution contained 0.3 g phloroglucinol in 10 ml absolute ethanol and mixed with 5 ml concentrated HCl (37%). The sample slices were filled with staining solution and covered for 5 min, followed by changing the staining solution with water. Calcofluor White and Auramine O staining The Phalaenopsis stems connected with the flower pedicel were collected and fixed with the fixative FAA. Samples were decolorized by alcohol dehydration and dissected in longitudinal sections using a blade. Tissue samples were mounted in ClearSee for one day and then stained with 0.1% Calcofluor White and 0.1% Auramine O (in ClearSee) overnight [52] . The tissue samples were washed in ClearSee for 2 h. Image acquisition was performed using an Olympus FV3000 confocal microscope (Nikon, Japan), and Calcofluor White used 405 nm excitation and was detected at 430–450 nm for cellulose (cyan color), while Auramine O used 488 nm excitation and was detected at 500–600 nm for lignin and cuticle (yellow color). Cryo-scanning electron microscopy The procedure used for Cryo-SEM was described in a previous study [6] . Briefly, the perianths were dissected and frozen using liquid nitrogen and transferred to the sample preparation chamber at −160 °C. The samples were etched for 10 min at −85 °C and were observed under a cryo-scanning electron microscope after gold coating (FEI Quanta 200 SEM, Quorum Cryo System PP2000TR FEI; FEI Company, Hillsboro, Oregon). FRET analysis The procedure used for FRET analysis was described in the previous studies [6] , [18] . 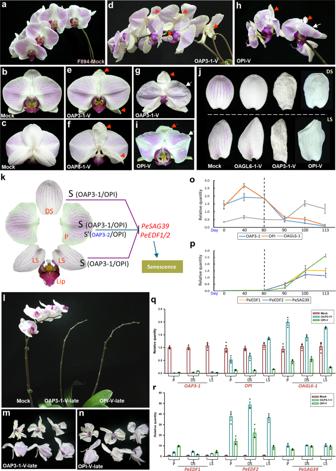Fig. 3: The OAP3-1 and OPI B functional proteins regulated sepal/petal senescence. a–cThe inflorescence (a), front view (b) and back view (c) of flowers of the control (Mock)PhalaenopsisF894.d–fThe inflorescence (d), front view (e) and back view (f) of flowers ofOAP3-1-VIGS F894, which showed early senescence of the sepals (red arrows).gThe senescence of theOAP3-1-VIGS petal (white arrow) occurred later than did that of the dorsal/lateral sepals (red arrow).h–iThe inflorescence (h) and front view (i) of flowers ofOPI-VIGS F894, which showed early senescence of the sepals (red arrow) and petals (white arrow).jThe dorsal (DS) and lateral (LS) sepals of control (Mock),OAGL6-1-VIGS,OAP3-1-VIGS, andOPI-VIGS F894 (from left to right) at the same stage.kSummary of the protein complexes that regulate sepal/petal senescence in orchid flowers. The OAP3-1/OPI B functional proteins may form a senescence complex (S), which is exclusively required for the suppression ofPeSAG39/PeEDF1/2expression and senescence in dorsal (DS) and lateral (LS) sepals. S and minor S’ (OAP3-2/OPI) complexes have complementary functions in regulating petal (P) senescence.l–nAt the same stage, all the flowers were senescent and abscised from theOAP3-1-VIGS-late (l, middle) (m) andOPI-VIGS-late (l, right) (n) inflorescences, whereas the flowers of the control (Mock) inflorescences showed no sign of senescence or abscission (l, left).o–pAnalysis of the expression profile forOAP3-1/OPI/OAGL6-1(o) andPeSAG39/PeEDF1/2(p) throughout flower development. The dashed lines indicate that the senescence of the F894 flowers starts at 80–90 days after flower opening. Error bars show ±SD.n= 3 biologically independent samples.q,rAnalysis of the expression ofOAP3-1/OPI/OAGL6-1(q) andPeSAG39/PeEDF1/2(r) in the petals (P), dorsal sepals (DS) and lateral sepals (LS) of control (Mock),OAP3-1-VIGS-late andOPI-VIGS-late F894 flowers. Error bars show ±SEM.n= 3 biologically independent samples. Source data underlying Fig. 3o–r are provided as a Source Data file. Briefly, to fuse OAGL6-1/OAP3-1/OAGL6-2/OAP3-2/OPI with CFP or YFP, the cDNAs for Phalaenopsis OAGL6-1/OAP3-1/OAGL6-2/OAP3-2/OPI were obtained by PCR amplification using gene-specific primers (Supplementary Table 3 ) and cloned into the pEpyon-36K and pEpyon-37K vectors upstream of the CFP or YFP sequence under the control of the CaMV 35S promoter. The above constructs were transformed into the Agrobacterium strain C58C1. Different ectopic proteins were expressed in tobacco leaf cells through Agrobacterium -infiltrated N. benthamiana leaves by being infiltrated in 10 mM MgCl2 at room temperature until immersed. A confocal microscope was used to detect the fluorescence signals in the nucleus. The procedure used to visualize fluorophores was described in a previous study [9] . Briefly, an Olympus FV1000 confocal microscope (Olympus FV1000, Tokyo, Japan) and the soft FV-ASW 3.0 software were used to visualize fluorophores and to calculate the raw FRET and FRET efficiency values. The mean value of FRET efficiency in the nucleus was calculated to evaluate the variation in protein interaction distances among different protein complexes ( n > 4). Virus-induced gene silencing experiment Since two DNA fragments in different independent nonconserved regions used for each of the OAGL6-2 -VIGS, OAGL6-1 -VIGS, OAP3-1 -VIGS, OAP3-2 -VIGS, OPI- VIGS, PeMYB12 -VIGS, and PeMYB11- VIGS experiments generated the similar mutant phenotypes (Supplementary Figs. 13 – 19 ), we thus used one specific DNA fragment for each target gene in subsequent VIGS experiments. To ensure the specificity of VIGS silencing effects for each target gene, DNA fragments contained the sequences specific for OAGL6-1 (PeMADS10), OAGL6-2 (PeMADS9), OAP3-1 (PeMADS2), OAP3-2 (PeMADS3) , and OPI (PeMADS6) in the highly variable C-terminal region (Supplementary Figs. 20 , 21 ), and for PeMYB12 and PeMYB11 , the variable regions located downstream from the highly conserved R2R3 MYB DNA-binding domain (Supplementary Fig. 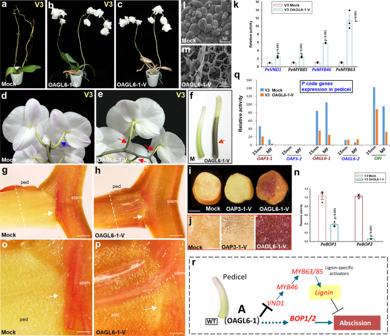Fig. 4: The OAGL6-1 protein regulated pedicel abscission in orchids. a,bThe flowers were senescent and abscised completely from the control (Mock) inflorescence (a), whereas senescent flowers were not abscised from theOAGL6-1-VIGS inflorescence (b) ofPhalaenopsisV3.cThe senescent flowers were still not abscised three months after the plant (b) had completely dried.d–fThe back views of flowers of the control (Mock) (d) andOAGL6-1-VIGS (e)PhalaenopsisV3. A dark brown color was observed in the pedicel ofOAGL6-1-VIGS (red arrow in (e,f)) but was absent in the control (Mock) pedicel (blue arrow in (d)) (f).g–hThe longitudinal views for pedicels (ped) and the connected stems of the control (Mock) (g)andOAGL6-1-VIGS V3 (h) after staining by phloroglucinol. The arrows indicate the AZ in the junction of the pedicel and stem. The dashed lines indicate the place used for the cross view in (i,j). Bars = 1 mm.iCross view of the pedicels of the control (Mock),OAP3-1-VIGS andOAGL6-1-VIGS V3 (from left to right) after staining by phloroglucinol. Bars = 1 mm.jClose-up image of the phloroglucinol-stained pedicels from (i). Bars = 100 µm.k,nAnalysis of the expression levels ofPeVND1,PeMYB85,PeMYB46, andPeMYB63(k) as well asPeBOP1andPeBOP2(n) in the pedicels of control (Mock) andOAGL6-1-VIGS V3 flowers. Error bars show ±SEM.n= 3 biologically independent samples. Thepvalue indicates significant differences from the control (Mock) value. The statistical test used was two-sided according to Student’st-test.l,mSEM image of pedicel AZs in control (Mock) (l) andOAGL6-1-VIGS (m) V3 flowers. Bars = 50 µm.o,pClose-up of the phloroglucinol-stained junctions for the pedicel (ped) and the stem of the control (Mock) (o) andOAGL6-1-VIGS V3 (p) from (g,h). The arrows indicate the AZ region with the small differentiated cells formed. The cells in the AZ region in (p) were altered by the penetration of lignin from the pedicel to the stem. Bars = 300 µm. In (j,l,m,o,p), each experiment was repeated twice independently with similar results.qAnalysis of the expression levels ofOAP3-1,OAP3-2,OAGL6-1,OAGL6-2, andOPIin 15 mm and mature flower pedicels of control (Mock) andOAGL6-1-VIGS V3 flowers. The data were derived from one NGS data.rIn wild-type orchid flowers, OAGL6-1 proteins may form an abscission complex (A) to promote the abscission of pedicels by suppressing the expression ofVND1/MYB46/63/85and lignin formation and to ensure the normalBOP1/2expression and subsequent AZ formation. Source data underlying Figs. 4k, 4n, and 4q are provided as a Source Data file. 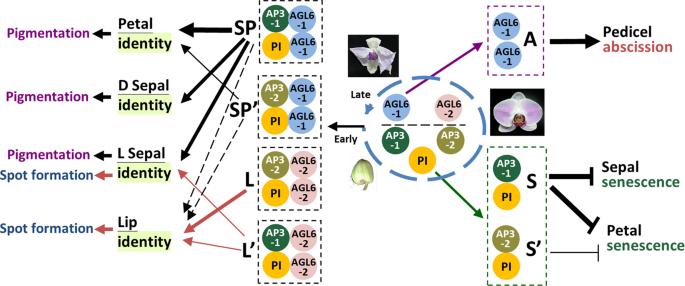Fig. 5: The multifunctional evolution of P-code genes in orchids. In orchids, twoAGL6(OAGL6-1,-2), twoAP3(OAP3-1,-2) and onePI(OPI) gene play key roles (blue dashed circle) in regulating perianth identity and other developmental processes in flowers. During early flower initiation, the L (OAP3-2/OAGL6-2/OPI) complex determines the lips, whereas the SP (OAP3-1/OAGL6-1/OPI) complex determines sepal/petal identity. In addition, an L’ complex (OAP3-1/OAGL6-2/OPI) is also likely involved in regulating the lips and lower parts of the lateral sepal identity/morphology, whereas an SP’ complex (OAP3-2/OAGL6-1/OPI) is likely involved in regulating the petal and lip identity/morphology. After flower organ identity has been determined, SP/SP’ complexes have an additional function in positively regulating (black arrow→) anthocyanin accumulation and pigmentation in sepals/petals, whereas L’/L complexes can regulate (red arrow→) red spot formation in lateral sepals and lips. During flower development, the OAP3-1/OPI B class proteins from the SP complex could form a separate senescence complex (S) to suppress (⊣) the senescence of the sepal/petal in orchids. An S’ complex (OAP3-2/OPI/X) with minor complementary function for the S complex could suppress (⊣) petal senescence. The orchid OAGL6-1 from the SP complex may form an abscission complex (A) to ensure (→) the abscission of the pedicel from senescent flowers during the late stage of flower development. AGL6-1: OAGL6-1, AGL6-2: OAGL6-2, AP3-1: OAP3-1, AP3-2: OAP3-2, PI: OPI. 22 ) were obtained by PCR amplification using gene-specific primers (Supplementary Table 4 ) and were inserted into the VIGS vector pCymMV-Gateway [53] . The att B sites (sequences in bold letters in Supplementary Table 3 ) were for in vitro recombination with att P sites in the VIGS vector pCymMV-Gateway to generate recombinant clones using Gateway ® BP Clonase II Enzyme Mix (Invitrogen™, Life Technologies, Carlsbad, CA, USA). pCymMV-Gateway-OAGL6-1, pCymMV-Gateway-OAGL6-2, pCymMV-Gateway-OAP3-1, pCymMV-Gateway-OAP3-2, pCymMV-Gateway-OPI, pCymMV-Gateway-PeMYB12, pCymMV-Gateway-PeMYB11 and the empty pCymMV-Gateway as a control were transformed into Agrobacterium tumefaciens EHA105 for further inoculation. The leaf infiltration experiments in Phalaenopsis orchids were performed as described previously [6] , [54] . Briefly, suspensions were injected into the leaf just above the site where the inflorescence emerged. At least three plants were inoculated with each pCymMV-Gateway construct for every infiltration. Flower samples were collected and analyzed at 45 DPI (days post inoculation), when the last bud of the Phalaenopsis inflorescences bloomed. The total number of VIGS experiments and plants analyzed for OAGL6-1 (PeMADS10), OAGL6-2 (PeMADS9), OAP3-1 (PeMADS2), OAP3-2 (PeMADS3), OPI (PeMADS6), PeMYB12 , and PeMYB11 in three different varieties of Phalaenopsis orchids are listed in Supplementary Tables 5 – 7 . Reporting summary Further information on research design is available in the Nature Research Reporting Summary linked to this article.